The landscape of viral expression and host gene fusion and adaptation in human cancer Viruses cause 10–15% of all human cancers. Massively parallel sequencing has recently proved effective for uncovering novel viruses and virus–tumour associations, but this approach has not yet been applied to comprehensive patient cohorts. Here we screen a diverse landscape of human cancer, encompassing 4,433 tumours and 19 cancer types, for known and novel expressed viruses based on >700 billion transcriptome sequencing reads from The Cancer Genome Atlas Research Network. The resulting map confirms and extends current knowledge. We observe recurrent fusion events, including human papillomavirus insertions in RAD51B and ERBB2 . Patterns of coadaptation between host and viral gene expression give clues to papillomavirus oncogene function. Importantly, our analysis argues strongly against viral aetiology in several cancers where this has frequently been proposed. We provide a virus–tumour map of unprecedented scale that constitutes a reference for future studies of tumour-associated viruses using transcriptome sequencing data. A century of tumour virology has revealed that seven types of viruses cause 10–15% of all human malignancies [1] . Viruses can cause cellular transformation by expression of viral oncogenes, by genomic integration to alter the activity of cellular proto-oncogenes or tumour suppressors, and by inducing inflammation that promotes oncogenesis. Viral aetiology is particularly evident in cervical carcinoma (CESC), which is almost exclusively caused by high-risk human papillomaviruses (HPV), and in hepatocellular carcinoma (LIHC), where infection with hepatitis B virus (HBV) or hepatitis C virus (HCV) is the predominant cause in some countries [2] . In addition, several rare cancers have a strong viral component, including Epstein–Barr virus (EBV)/human herpes virus (HHV) 4 in most Burkitt’s lymphomas. Huge advances in the prevention of virus-associated cancer has been made through vaccination programmes against HPV and HBV, second only to smoke cessation in the number of yearly cancer cases prevented worldwide [3] . Our current knowledge of virus–tumour associations is based largely on data gathered with low-throughput methodologies in the pre-genomic era. However, massively parallel sequencing is now showing promise for efficient unbiased detection of viruses in tumour tissue. This recently led to the discovery of a new polyomavirus as the cause of most Merkel cell carcinomas [4] , where essential virus–host interactions are currently being targeted in clinical drug trials [5] . Recent studies describe techniques for detection of viruses using high-throughput RNA or DNA sequencing [6] , [7] , and massively parallel sequencing has been used to survey sites of genomic integration of HBV in hepatocellular carcinoma [8] , [9] . Similarly, viral integration sites were recently mapped in 17 cervical and 239 head and neck carcinomas by detecting host–virus fusions in transcriptome sequencing (RNA-seq) data from The Cancer Genome Atlas (TCGA) [10] . These studies provided important insights and clearly demonstrate the potential of the methodology, but the scope and the number of tumours has thus far been limited. This motivates a broad unbiased survey of viral expression and integration in human cancer. Here we screen for expressed viruses in a diverse landscape of human cancer, encompassing 19 tumour types and 4,433 tumours, using RNA-seq data generated within the TCGA consortium. The resulting map provides a cross-cancer view of tumour–virus associations on a previously unseen scale and level of detail, and enables several powerful analyses. Our observations fall into six main categories: confirmation of established associations, such as high-risk HPV in cervical and head and neck cancer, which validates our methodology and provides reference viral expression levels and patterns in tumours with known viral aetiology; confirmation or rejection of controversial hypotheses, such as HPV18 in colorectal cancer; rare occurrences of known viruses in novel contexts; new viral isolates, including a novel recombinant enterovirus strain; novel recurrent host—virus fusion events, such as HPV insertions in ERBB2 and RAD51B ; and patterns of coadaptation between viral and host gene expression. A map of tumour viruses in 19 human cancers We used two complementary approaches to detect and quantify expression of known and novel viruses in tumours ( Fig. 1a , Methods). Briefly, RNA-seq libraries were filtered of human content, and remaining sequences were screened for matches to the complete RefSeq collection of viral genomes ( n =3,590 excluding bacteriophages). Viral mRNA was quantified by computing the fraction of viral reads (FVR), presented as parts per million (p.p.m.) of total library size. To enable detection of missing strains and novel viruses, we de novo assembled non-human reads into contiguous segments (contigs) that were annotated while allowing for strong sequence divergence. On the basis of this, we added additional viral genomes, such as papilloma types missing in RefSeq and two novel assembled genomes ( Supplementary Table S1 and Supplementary Fig. S1 ), to allow quantification as described above. Cases with unnaturally restricted viral genomic read coverage, probably due to traces of recombinant DNA, were excluded (Methods). 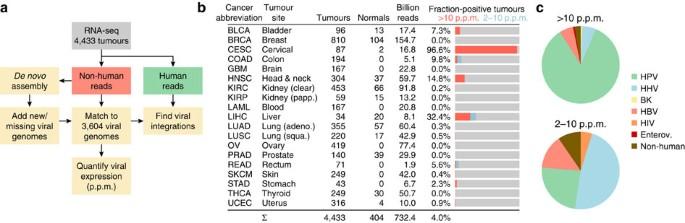Figure 1: Unbiased detection of viral expression in 4,433 tumours. (a) Analysis pipeline. Non-human reads were matched to a database of 3,590 RefSeq viral genomes, that was complemented with 12 additional known and 2 partial novel genomes detected byde novoassembly of viral reads. (b) Included cancer types and statistics. Bar graphs show fraction of tumours with strong viral expression (>10 p.p.m. viral reads in library) as well as weaker detections (2–10 p.p.m.). (c) Relative numbers of positive tumours for major virus categories, with strong and weak detections shown separately. Figure 1: Unbiased detection of viral expression in 4,433 tumours. ( a ) Analysis pipeline. Non-human reads were matched to a database of 3,590 RefSeq viral genomes, that was complemented with 12 additional known and 2 partial novel genomes detected by de novo assembly of viral reads. ( b ) Included cancer types and statistics. Bar graphs show fraction of tumours with strong viral expression (>10 p.p.m. viral reads in library) as well as weaker detections (2–10 p.p.m.). ( c ) Relative numbers of positive tumours for major virus categories, with strong and weak detections shown separately. Full size image We applied our pipeline to RNA-seq libraries from 19 cancers, encompassing a total of 4,433 tumours and 404 normal tissue controls that were each sequenced at an average depth of 151 million reads ( Fig. 1b ; additional library and sample information in Supplementary Table S2 ). We identified 178 tumours with FVR (viral expression) >2 p.p.m., but found that most positive cases had considerably higher levels (on average 168 and up to 854 p.p.m. ; the complete results are available in Supplementary Data 1 ). Expectedly, CESC and LIHC showed the highest proportion of virus-positive tumours (96.6% and 32.4%, respectively, >2 p.p.m. ), followed by head and neck squamous cell carcinoma (HNSC, 14.8%; Fig. 1b ). De novo assembly revealed HPV in 15/18 CESC tumours that were originally negative, demonstrating a high sensitivity for detecting missing and novel viruses. Comparison with HPV status as determined by in situ hybridization in HNSC showed that 8/8 positive and 44/44 negative samples were correctly classified by our pipeline. The known tumour viruses HPV and HBV constituted the vast majority of strong signals >10 p.p.m. (90.5%; Fig. 1c ). In contrast, matches in the 2–10-p.p.m. range were often because of HHVs that are known to infect and remain latent in lymphocytes (47.6%). Many of these detections could be attributed to cytomegalovirus (CMV/HHV5) and EBV in colon adenocarcinoma (COAD), probably because of lymphocytic infiltration ( Fig. 2a ). T-lymphocyte infiltration could also probably explain one case of low-FVR HIV1 in rectal adenocarcinoma (READ). We conclude that viruses that are actively participating in tumour formation and maintenance often, but not always, show FVR values >10 p.p.m. 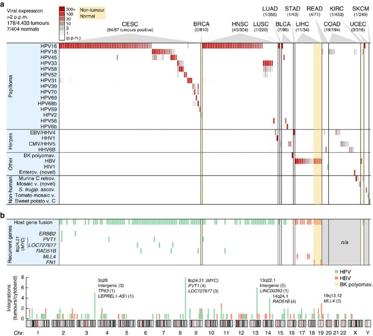Figure 2: RNA expression and host–virus fusion for 28 viruses detected in 178 tumours. (a) RNA-seq-derived expression levels for 28 viruses (vertical axis) detected at >2 p.p.m of total library reads in at least one tumour, across 178 virus-positive tumours from 19 cancer types (horizontal axis). Viruses identified only because of sequence similarity with related strains were not included. (b) In addition to viral gene expression, genomic viral integration may have functional consequences. A large fraction of positive tumours identified inacarried viral integrations (top row), as evidenced by host–virus fusion transcripts in paired-end RNA-seq. Some genes showed recurrent integration in multiple tumours (six bottom rows). Integrations were quasi-randomly distributed across the genome (bottom chromosome plot) with some preferred loci. Select genes are shown for cytobands with recurrent integrations (number of tumours in parentheses). n/a, no paired-end data available. Figure 2: RNA expression and host–virus fusion for 28 viruses detected in 178 tumours. ( a ) RNA-seq-derived expression levels for 28 viruses (vertical axis) detected at >2 p.p.m of total library reads in at least one tumour, across 178 virus-positive tumours from 19 cancer types (horizontal axis). Viruses identified only because of sequence similarity with related strains were not included. ( b ) In addition to viral gene expression, genomic viral integration may have functional consequences. A large fraction of positive tumours identified in a carried viral integrations (top row), as evidenced by host–virus fusion transcripts in paired-end RNA-seq. Some genes showed recurrent integration in multiple tumours (six bottom rows). Integrations were quasi-randomly distributed across the genome (bottom chromosome plot) with some preferred loci. Select genes are shown for cytobands with recurrent integrations (number of tumours in parentheses). n/a, no paired-end data available. Full size image Importantly, we note an absence of relevant viral expression in several cancers otherwise subject to regular speculation about strong viral aetiology, including EBV in breast invasive carcinoma and CMV in glioblastoma multiforme [11] , [12] . The deep sequencing depth in these samples allowed us to safely estimate upper limits on viral expression: in the worst-case tumours, CMV was expressed at <0.05 p.p.m. in glioblastoma multiforme and EBV at <0.09 p.p.m. in breast invasive carcinoma ( P =0.01, binomial distribution). These results, in combination with large samples (167 and 810 tumours, respectively), argue strongly against viral aetiology, although rare involvement cannot be excluded. Papillomavirus prevalence across cancers Overall occurrences of HPV agreed closely with current knowledge: CESC showed 96.6% association with HPV, similar to recent large surveys [13] ( Fig. 2a ). No other viruses were found in CESC, further supporting that detections were highly specific. Twelve HPV types, all previously described as associated, were found in 84 positive cervical tumours, with HPV16 and HPV18 expectedly being predominant (65.5% and 13.1% of positive cases, respectively). HNSC showed 14.1% HPV association, with 83.7% and 14.0% of positive tumours attributed to HPV16 and HPV33, respectively; this is notably different from CESC and compatible with earlier data [14] . Less common but previously observed associations included HPV6b and high-risk types in bladder urothelial carcinoma (BLCA), and HPV16 in lung squamous cell carcinoma (LUSC) and uterine endometroid carcinoma (UCEC). HPV typically showed prominent expression, with FVR values up to 848 p.p.m. (>140.000 reads) but more typically in the 100–200-p.p.m. range ( Fig. 3a ). 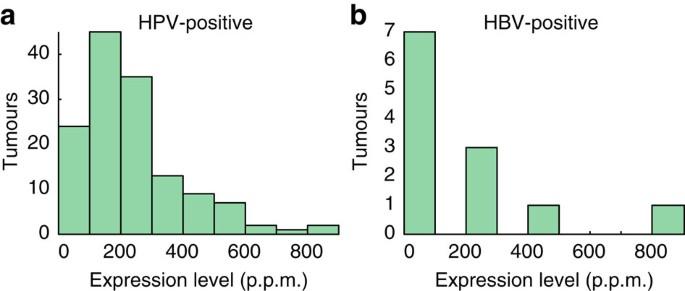Figure 3: Distribution of viral expression levels across HPV- and HBV-positive tumours. The histograms show viral expression levels (FVR) for 138 HPV-positive (a) and 12 HBV-positive (b) tumours in 100-p.p.m. intervals. Figure 3: Distribution of viral expression levels across HPV- and HBV-positive tumours. The histograms show viral expression levels (FVR) for 138 HPV-positive ( a ) and 12 HBV-positive ( b ) tumours in 100-p.p.m. intervals. Full size image There has been controversy regarding associations between HPV and colorectal cancer, with prevalence ranging from 0 to 83% in different studies [15] , [16] . Contamination has been suggested as a possible cause of false positives [16] . We observed weak expression (2–6.5 p.p.m.) of HPV18 in 5 cases (1.9%) of COAD/READ, which increased to 12 cases (4.5%) with inclusion of the 1–2-p.p.m. range ( Supplementary Data 1 ). Viral gene expression patterns in these samples were different from known HPV-induced tumours, with consistent expression of E1 more indicative of active replication ( Supplementary Fig. S2 ). We did not detect HPV18 in other tumours apart from CESC, which argues against contamination. HPV18 is one of few HPV types with glandular tropism [17] , and could conceivably infect colorectal adenocarcinomas. We conclude that earlier reports of HPV18 in colorectal tumours are probably correct. However, prevalence may have been overestimated, and expression patterns and levels speak against a contribution to carcinogenesis. Apart from matched normal liver samples with expected HBV (discussed below), only 2/404 normal tissue controls tested positive in this study, both with papillomavirus ( Fig. 2a ): one breast biopsy with low levels (3.1 p.p.m.) of a wart virus, HPV2, which expressed early as well as late genes indicative of active production of viral particles, and a normal kidney sample with HPV18 (12.9 p.p.m. ), with viral gene expression similar to HPV in COAD/READ consistent with productive viral infection ( Supplementary Fig. S2 ) but also with evidence of host–virus fusion ( Fig. 2b , fusions are discussed below). These cases suggest novel tropisms for HPV, but more work is needed. Hepatitis virus prevalence As expected, HBV was detected in hepatocellular cancer ( Fig. 2a ): 11/34 (32.3%) of LIHC tumours expressed HBV at up to 854 p.p.m., but more typically in the 2–100-p.p.m. range ( Fig. 3b ). In positive cases, we consistently detected HBV in matched normal liver controls (5/5). A single tumour expressed HCV but at low levels (0.8 p.p.m. ; Supplementary Data 1 ), likely explained by the non-polyadenylated nature of the HCV genome [18] . No other viruses were detected in LIHC. Inflammation/cirrhosis is a major promoter of HBV-induced oncogenesis, but expression of the viral gene X ( HBx ) also contributes [19] . Consistently, HBx was the predominantly expressed viral gene ( Supplementary Fig. S3 ). In addition to LIHC, we found a single clear cell renal cell carcinoma (KIRC) primary tumour with moderate expression (28.9 p.p.m.) of the common HBV genotype C ( Fig. 2a , Supplementary Table S3 ). However, although viral genes were expressed similarly to HBV-positive LIHC tumours ( Supplementary Fig. S3 ) and the tumour mRNA profile was similar to other KIRC samples, further analysis revealed weak but consistent induction of LIHC marker genes in this sample ( Supplementary Fig. S4 ). This supports that low-grade contamination with LIHC RNA could explain this detection. Rare occurrences and novel viral sequences BK polyomavirus (BKV) infects kidneys and the urinary tract, and has been implicated as a human tumour virus because of its oncogenic large tumour antigen ( TAg ) gene. There are contrasting reports of BKV in bladder cancer, ranging from high frequency to no association or lack of TAg expression [20] . We detected abundantly expressed BKV (318 p.p.m.) in 1/96 BLCA tumours, with predominant expression of full-length large TAg ( Supplementary Fig. S5 ) as well as evidence of host–virus fusion ( Fig. 2b , fusions are discussed below). This gives additional support for an aetiological role for BKV in rare cases of bladder cancer. HHV1, which normally causes mucoepithelial herpes lesions [21] , was detected at high FVR (338 p.p.m.) in a single HNSC tumour ( Fig. 2a ). HHV1 has not been described in tumours, although elevated HHV1 antibody titres have been shown in HNSC patients [22] . High HHV1 mRNA in this tumour could reflect reactivated virus infecting adjacent epithelium rather than tumour tissue. Enteroviruses cause a range of diseases including gastroenteritis. De novo assembly in COAD detected a novel enterovirus, revealed by detailed analysis as a recombinant of Coxsackievirus strains A19 and A22 ( Supplementary Fig. S1 ). Presence of the virus in tumour tissue is supported by high FVR (67.0 p.p.m.) and the vast tropism of Coxsackieviruses [21] . Although our analysis involved unbiased matching to 3,065 non-human viral genomes, only a few hits involved viruses unlikely to infect humans (7/4,837 samples, Fig. 2a ). One COAD tumour showed strong (456 p.p.m.) expression of murine type C retrovirus, also detected at low levels (3.1 and 3.8 p.p.m.) in another COAD tumour and a normal kidney biopsy. Murine type C retrovirus has strong similarity to XMRV, which was erroneously associated with disease because of contamination from common murine cell lines [23] . De novo assembly detected a novel mosaic-like virus ( Supplementary Fig. S1 ) in COAD, and traces of tomato mosaic virus (3.6 p.p.m.) were found in one uterine endometroid carcinoma tumour. These viruses, and two other non-human detections ( Fig. 2a ), are unlikely to be oncogenic pathogens, suggesting contamination or environmental exposure at the tumour site. Analysis of host–virus fusions HPV genomic integrations are believed to occur as a consequence of HPV oncogene-induced chromosomal instability, and integrations in or near known tumour genes have been described, sometimes in conjunction with local copy-number change and altered expression of targeted genes [24] , [25] , [26] . Integrations associated with altered gene activity are similarly important in HBV-induced oncogenesis [8] . We employed a stringent procedure for detecting integrations as evidenced by host–virus fusion transcripts in RNA-seq, considering only breakpoints supported by multiple discordant sequencing mate pairs where human reads clustered within a limited region (Methods). We validated our methodology using whole-genome sequencing data from nine HPV-positive HNSC tumours, and found that eight of nine RNA-seq-derived integrations had support from discordant mate pairs in whole-genome sequencing libraries ( Supplementary Table S4 ). Confirming previous data [25] , we observed a high integration frequency for HPV18 (100%) and a lower frequency for HPV16 (58.5%; Fig. 2b , Supplementary Data 2 ). Similarly, confirmatory, most HBV-positive tumours and normal tissue controls had viral integration [8] (76.5%), and all HHV cases lacked integration ( Fig. 2b ). Both HPV and HBV integrations were widespread across the genome, with a few hotspots of recurrent integration ( Fig. 2b ). Further analysis in HNSC revealed the positional distribution to be non-random with a strong preference for integration near DNA copy-number breakpoints. A large fraction of integration clusters (41.8%) colocalized (<10 kb, close to the copy-number mapping resolution) with a segment boundary, supporting that integrations could have a widespread effect on local genomic instability in HNSC ( Fig. 4 , P <1e−8, randomization test). 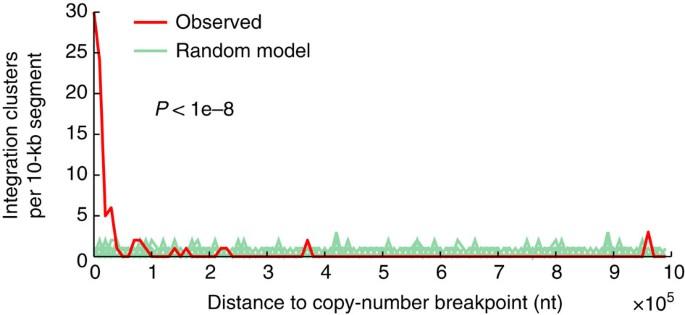Figure 4: Integrations in HNSC colocalize with DNA copy-number breakpoints. One hundred and ten HPV integration clusters (31 unique integrations) were compared with copy-number breakpoints determined using segmented Affymetrix SNP6 microarray data from TCGA. The distance to the nearest breakpoint was calculated for each cluster, and the observed distribution was tested for non-random colocalization by comparing with a uniform random integration model (P<1e−8 based on 1e−8 randomizations; 100 shown). Integration clusters (41.8%) were within 10 kb, whereas the random expectation was <0.5%. Ten kilobases are close to the SNP6 mapping resolution (average probeset spacing ~3 kb). Figure 4: Integrations in HNSC colocalize with DNA copy-number breakpoints. One hundred and ten HPV integration clusters (31 unique integrations) were compared with copy-number breakpoints determined using segmented Affymetrix SNP6 microarray data from TCGA. The distance to the nearest breakpoint was calculated for each cluster, and the observed distribution was tested for non-random colocalization by comparing with a uniform random integration model ( P <1e−8 based on 1e−8 randomizations; 100 shown). Integration clusters (41.8%) were within 10 kb, whereas the random expectation was <0.5%. Ten kilobases are close to the SNP6 mapping resolution (average probeset spacing ~3 kb). Full size image It is noteworthy that of six genes with recurrent integrations, all were known cancer genes or previously described recurrent targets ( Fig. 2b ; detailed fusion sites are presented in Supplementary Table S5 ). The MYC region on chromosome 8q24.21 is a known site of frequent HPV integration in CESC [24] , and consistently we observed seven tumours with breakpoints in the PVT1 and LOC727677/RP11-382A18.1 long non-coding RNAs (lncRNAs), downstream and upstream of MYC , respectively. Although ERBB2 / HER2 contribution to cervical cancer has been controversial, it is known that the HPV16 E6 protein can stabilize ErbB2 (ref. 27 ). HPV16, but not HPV18, integrated in ERBB2 in two CESC tumours, supporting that HPV might have a dual role in activating and stabilizing ERBB2 in a subset of samples. Repeated HPV integrations (four tumours) were seen in the RAD51 paralogue RAD51B ( RAD51L1 / REC2 ) on chromosome 14q24.1, in one case in-frame with the HPV E6 gene ( Supplementary Fig. S6 ). 14q24 is a known fragile region and weakly preferred integration site [26] , but recurrent integration specifically in RAD51B has not been described. Retinoblastoma protein (RB) inhibition increases RAD51B-induced apoptosis and the two proteins interact [28] , suggesting that RAD51B inactivation by HPV integration could act synergistically with the HPV E7 gene, which inactivates RB. Similarly, 13q22 is a weakly preferred fragile site [26] where we observed a relatively high frequency of integration (six tumours), specifically in 13q22.1 near the LINC00393 lncRNA ( Fig. 2b ). Results from LIHC confirmed recurrent HBV fusions with MLL4 and FN1 in tumours and adjacent normal liver, respectively [8] , two of which were found to be in-frame ( Supplementary Fig. S6 ). We next investigated the relationship between expression and integration for recurrent genes by comparing tumours with and without integration. Most genes showed altered mean expression, although there were exceptions for individual tumours. Of two tumours with strong ERBB2 transcriptional induction in CESC, one had HPV integration in this gene ( Fig. 5a ). The PVT1 and LOC727677 lncRNAs, in the MYC region, had significantly higher expression in tumours with integration. RAD51B showed a weak, non-significant, reduction in tumours with HPV integration. Consistent with previous data [8] , MLL4 was strongly induced in LIHC samples with HBV integration, whereas FN1 was not significantly altered ( Fig. 5b ). Although normal control samples are limited in TCGA, we identified nine cases of gene integration with an available matched normal lacking integration ( Supplementary Fig. S7 ). Five of nine cases showed strong (more than fourfold) induction in the tumour compared with the normal control, including MLL4 (6.0-fold). Our results support that the activity of tumour genes can be altered by viral insertions, and nominate ERBB2 and RAD51B as functional targets. 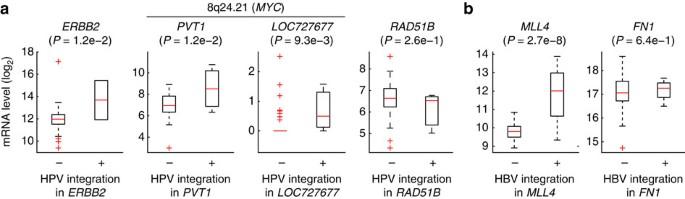Figure 5: Fusion is associated with altered expression of recurrent target genes. (a) Expression levels ofERBB2(n=2),PVT1(n=3),LOC727677(n=3) andRAD51B(n=3) were typically altered in CESC tumours with HPV integration, as evidenced by host–virus fusion.P-values were calculated using Student’st-test. (b) Similar toa, but for LIHC samples with and without HBV integration inMLL4(n=3) andFN1(n=2). In the box plots, the central mark is the median and the box edges are the 25th and 75th percentiles. Figure 5: Fusion is associated with altered expression of recurrent target genes. ( a ) Expression levels of ERBB2 ( n =2), PVT1 ( n =3), LOC727677 ( n =3) and RAD51B ( n =3) were typically altered in CESC tumours with HPV integration, as evidenced by host–virus fusion. P -values were calculated using Student’s t -test. ( b ) Similar to a , but for LIHC samples with and without HBV integration in MLL4 ( n =3) and FN1 ( n =2). In the box plots, the central mark is the median and the box edges are the 25th and 75th percentiles. Full size image Coadaptation between virus and host mRNA expression Our comprehensive virus–tumour map provided further opportunities to investigate the interplay between viruses and host mRNA expression, both within and across tumour types. The HPV genome contains the viral oncogenes E6 and E7 that inactivate p53 and RB, respectively, as well as E5 that may also promote carcinogenesis [29] . DNA microarray studies [30] , [31] , [32] have previously revealed that HPV-positive versus HPV-negative tumours express differential sets of transcription factors and cell cycle regulators (for example, cyclins E/B versus D/A, respectively), and that the transcriptional differences seem to largely be direct consequences of HPV oncogene action. The 42/262 HPV-positive/-negative HNSC tumours included in our survey enabled a more powerful set-up for studying HPV-induced mRNA changes, with the additional benefit of precise measurements from deep RNA-seq (on average 175 M reads per sample). Five hundred and ninety-seven host genes were at least fourfold induced or repressed based on the ratio of their median expression levels in HPV-positive compared with HPV-negative HNSC tumours ( q <0.05, false discovery rate based on Student’s t -test; Fig. 6a , Supplementary Data 3 ). Another 1,897 genes were altered above twofold ( q <0.05), showing that HPV has a more widespread impact on host gene expression than described previously. CDKN2A / P16-INK4A , widely used as a surrogate marker for HPV infection because of its induction upon RB inactivation by E7 (ref. 33 ), was among the most strongly induced genes (10.6-fold). Several additional cell cycle regulators and oncogenes showed prominent induction, including CDKN2C and MYB ( Fig. 6a ). Although gene set enrichment analysis (GSEA) [34] revealed highly significant overlaps with earlier studies [30] , [31] , most genes had not previously been associated with HPV status. This included MYCN (4.3-fold induced), normally not linked to HNSC progression but thus potentially important in HPV-induced oncogenesis. 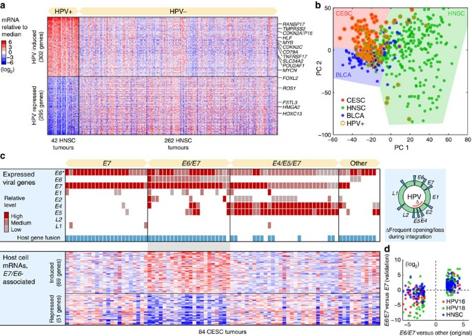Figure 6: Host gene expression and virus–host coadaptation. (a) Five hundred and ninety-seven host genes were associated with HPV status in HNSC, at a false discovery rate (q)<0.05 and with an absolute log2median expression ratio >2. Known cancer genes in the Cancer Gene Census47are indicated. The colour code indicates log2-transformed mRNA levels relative to the overall median. (b) PCA analysis of tumour mRNA expression profiles in CESC, HNSC and BLCA. Although there were systematic expression differences between cancer types, HPV-positive tumours clustered together regardless of type. (c) HPV-positive CESC tumours were subdivided by their viral gene expression patterns:E7-,E6/E7- andE4/E5/E7-expressing tumour subsets were tested for differential expression of host genes relative to remaining samples. One hundred and twenty host genes were differentially expressed in theE6/E7subset, using criteria described above. (d) Validation of theE6/E7signature. Most of the 120 genes were consistently induced/repressed inE6/E7compared withE7samples, also when only considering HPV16 (red)- or HPV18 (green)-positive tumours. In addition, most genes in the signature showed consistent expression changes in HNSCE6/E7compared withE6tumours (blue).E6*, truncated and probably non-functionalE6open reading frame. Figure 6: Host gene expression and virus–host coadaptation. ( a ) Five hundred and ninety-seven host genes were associated with HPV status in HNSC, at a false discovery rate ( q )<0.05 and with an absolute log 2 median expression ratio >2. Known cancer genes in the Cancer Gene Census [47] are indicated. The colour code indicates log 2 -transformed mRNA levels relative to the overall median. ( b ) PCA analysis of tumour mRNA expression profiles in CESC, HNSC and BLCA. Although there were systematic expression differences between cancer types, HPV-positive tumours clustered together regardless of type. ( c ) HPV-positive CESC tumours were subdivided by their viral gene expression patterns: E7 -, E6 / E7 - and E4 / E5 / E7 -expressing tumour subsets were tested for differential expression of host genes relative to remaining samples. One hundred and twenty host genes were differentially expressed in the E6 / E7 subset, using criteria described above. ( d ) Validation of the E6 / E7 signature. Most of the 120 genes were consistently induced/repressed in E6 / E7 compared with E7 samples, also when only considering HPV16 (red)- or HPV18 (green)-positive tumours. In addition, most genes in the signature showed consistent expression changes in HNSC E6 / E7 compared with E6 tumours (blue). E6 *, truncated and probably non-functional E6 open reading frame. Full size image To address whether HPV invokes similar effects in different cancer types, we performed principal components analysis of mRNA profiles from CESC, HNSC and BLCA tumours. Interestingly, although each tumour type expectedly was associated with a distinct expression signature, HPV infection status had an even greater impact on the transcriptome, as positive tumours tended cluster together regardless of type ( Fig. 6b ). This was confirmed by pairwise correlations: HPV-positive HNSC tumours were on average more similar to HPV-positive CESC tumours than HPV-negative HNSC tumours (Pearson’s r =0.054 and 0.041, respectively); remaining comparisons gave analogous results. This extends an earlier observation that many HPV-associated changes are shared between HNSC and CESC [31] . It is consistent with the widespread HPV-induced transcriptional effects described above, and notable considering the diverse tissue origins of these tumours. Having concluded that HPV has a dramatic impact on host transcription, we set out to investigate whether differential modes of viral gene expression and integration were associated with distinct host responses. Most HPV-positive tumours expressed E7 , consistent with previous expression and functional data pointing to E7 as the most potent HPV oncogene [35] , but also truncated E6 forms ( E6 *) that may lack full E6 activity ( Supplementary Fig. S8 , Supplementary Data 4 ). Remaining HPV oncogenes showed considerable inter-tumour diversity. We found that CESC HPV-positive tumours provided a suitable sample to study viral expression heterogeneity, and identified three major subsets based on relative levels: tumours expressing mainly E7 , E6 / E7 or E4 / E5 / E7 ( Fig. 6c ). E4 / E5 are typically lost during genomic integration [29] , and the fusion/integration frequency was consequently low in the E4 / E5 / E7 set while close to 100% in the other groups ( Fig. 6c ). We next tested the subsets for differential expression of host mRNAs relative to remaining samples. No host genes could be associated to the E7 or the E4 / E5 / E7 sets ( q <0.05), showing that neither genomic integration nor E4 / E5 expression has a strong impact on host expression. However, 69 and 51 host genes were induced or repressed at least fourfold, respectively, in the E6 / E7 subset ( q <0.05; Fig. 6c , Supplementary Data 5 ). Most genes in this signature were consistently induced/repressed in E6 / E7 compared with E6 samples based on HPV16 or HPV18 samples alone as well as in an independent cancer type (HNSC; Fig. 6d ), confirming them as robustly associated with E6 -expressing tumours. GSEA analysis revealed reduced expression of genes related to epithelium differentiation, epidermis development and previously defined markers of well-differentiated head and neck tumours ( q =9.3e−10, 7.3e−6 and 1.6e−3, respectively, false discovery rate based on a hypergeometric test) [36] . p53 exerts its tumour suppressive function not only by cell cycle arrest and apoptosis but also by restraining de-differentiation of mature cells [37] . The association of full-length E6 expression with a de-differentiated host signature could thus be mediated by its canonical inhibitory action on p53. Although HPV is known to induce host mRNA changes, our analysis shows that the detailed host response differs between tumours because of differential viral oncogene expression. In the present study, we used transcriptome sequencing data to generate a broad map of viral expression, as well as host gene fusion and interaction, in diverse human cancers. We introduce FVR as a robust quantitative metric for viral expression, but find that actual expression patterns also need to be considered to avoid false positives. Our unbiased map fits neatly with the overall model that has emerged from decades of low-throughput tumour virology, but also expands this model with several novel observations. Importantly, our results argue strongly against regular reports of high frequencies of HPV and other viruses in common cancers. Such findings may in part have arisen because of overly sensitive PCR-based assays, which may detect viral traces orders of magnitude lower than what we typically observe in virus-induced tumours (>10 p.p.m.). Viral integrations in CESC have not previously been assayed using massively parallel sequencing in comprehensive cohorts. Recurrent integrations, as evidenced by host–virus fusions, were typically in known cancer genes, including ERBB2, RAD51B and in the 13q22.1 intergenic region harbouring the LINC00393 lncRNA. Technical limitations of earlier methods may have caused these recurrent sites to be missed, as previously suggested for HBV [8] . Integrations were typically associated with altered gene expression, and our analysis in HNSC revealed strong association between viral integration and copy-number change, similar to what has been reported in CESC [38] . Although this is compatible with induction of local genomic instability, integration could alternatively be facilitated in these regions by pre-existing instability, and future studies should aim to better differentiate between these models. Analysis of host transcriptome perturbations caused by tumour virus proteins can facilitate identification and prioritization of cancer-causing genes and pathways [39] . Abundant RNA-seq data from hundreds of positive tumours here enabled us to analyse host gene expression in relation to viral infection and viral gene expression at a previously intractable scale and level of detail. The E6 / E7 -expressing subcategory of HPV tumours, which we could associate with a de-differentiated host signature, may be of particular interest. Future work should investigate this subtype in relation to mutational profiles, clinical variables and responsiveness to therapy. De novo assembly of novel viral sequences revealed an enterovirus recombinant and a new mosaic-like virus, and was highly efficient at identifying HPV when relevant strains were missing in our viral database. However, the number of discovered novel viruses was still surprisingly low. An exciting future application is rare cancers, which could lead more novel viruses or recurrent associations being uncovered. The present work provides a reference for expected viral expression levels in virus-induced tumours, and paves the way for future unbiased mapping of tumour-associated viruses in large-scale cancer genomics data sets. Detection of viruses in tumour RNA-seq RNA-seq data in BAM format for 19 cancers encompassing 4,433 tumours and 404 normal tissue controls was obtained from the TCGA CGHub repository (current data as of 25 February 2013). Unaligned (non-human) reads were extracted using bam2fastq ( http://www.hudsonalpha.org/gsl/information/software/bam2fastq ) and further filtered of human content using Bowtie [40] . The prinseq-lite utility [41] was used to remove low-complexity sequences (using a DUST threshold of 7) and short reads <45 nucleotides. Remaining reads were aligned to the RefSeq collection of viral genomes ( n =3,590 excluding bacterial phages), downloaded on 19 Dec 2012. For this, we used Bowtie, allowing up to 2 mismatches and a maximum of 25 alignments to the viral database. Before screening, the RefSeq viral genome database was complemented with additional missing genomes ( Supplementary Table S1 ) detected by de novo contig assembly described below. Alignment results were post-processed in Matlab (Mathworks Inc.) to generate detailed tables and reports. Viruses expressed >2 p.p.m. of total library reads are presented in Fig. 2 , whereas all detections >0.5 p.p.m. are documented in Supplementary Data 1 . A nearest-neighbor approach was applied to RNA-seq profiles to confirm the overall correctness of TCGA tissue annotations (98.2% correctly classified, Supplementary Data 6 ). We used low viral genomic read coverage (number of unique positions) as an indicator of unnaturally restricted expression. Manual inspection of such cases (<500 positions) led to the exclusion of several HHV5/CMV and human adenovirus C hits that were probably because of traces of recombinant DNA, including CMV promoter-containing plasmids ( Supplementary Data 7 contains graphical expression profiles for all positive tumours). We also filtered out artefactual matches to NC_008168.1, a budworm granulovirus, that were because of the presence of bacterial ribosomal RNA in several samples. HPV status for HNSC tumours determined by in situ hybridization was obtained from the TCGA repository. De novo viral genome assembly We used SOAPdenovo [42] , with a K-mer size of 25, for unbiased assembly of non-human reads, and considered contiguous segments (contigs) >400 nucleotides. To identify missing strains and novel viruses, contigs were matched to known viruses by BLAST [43] using a word size of 7. Simulated contigs from Merkel cell polyomavirus showed that the approach could detect unknown viruses with high sensitivity, also when considerably diverged from the reference genomes. On the basis of this analysis, we added additional viral genomes from other sources, such as papilloma types missing in RefSeq, as well as two novel assembled genomes ( Supplementary Fig. S1 and Supplementary Table S1 ). Post-processing included generation of html reports, describing all BLAST alignments >200 nucleotides. Identification of viral integration sites Sites of viral integration were identified using mate information from paired-end sequencing, similar in principle to a previous report [10] . Reads were subject to quality filtering as described above. Discordant human–viral mate pairs were identified by alignment of non-viral reads to the Hg19 human reference with Bowtie, allowing up to two mismatches and discarding non-uniquely mapped reads. Human mates in discordant pairs were clustered by position using a maximum gap size of 100. To identify single distinct breakpoints supported by multiple reads, we considered clusters with at least 10 reads (unique positions). Integrations into the mitochondrial genome, indicative of false positives, were completely absent at this level of stringency. Breakpoint clusters were finally annotated against the GENCODE (v11) gene annotation [44] . Recurrent integrations in TMPRSS3 were not considered, as they were due to a single long transcript likely to be a mis-annotation. For nucleotide-resolution mapping of integration breakpoints, we used the Subread aligner [45] to identify breakpoint-spanning reads that aligned in part to Hg19 and in part to the viral database. These were filtered based on the pair-end integration results, such that only those that aligned to relevant genes and viruses were considered. Breakpoints with support from at least 10 breakpoint-spanning reads were considered for further analysis. Host gene expression analyses Host gene expression analyses were done using TCGA Level 3 (RNASeqV2) transcription profiles. We tested for differential expression between HPV-positive/-negative tumours, and between subsets of tumours classified by their viral expression patterns, using Student’s t -test based on log 2 -transformed mRNA levels. We considered genes with detectable expression in at least half of the samples. Expression ratios were computed by comparing median levels in each group. P- values were corrected for multiple testing by computing q -values (false discovery rates) as described previously [46] . Viral genes were manually classified as having high, medium, low or absent relative expression based on read density plots ( Supplementary Fig. S8 and Supplementary Data 4 ). PCA analysis was performed based on 14,714 genes with expression level >500 in at least one sample. How to cite this article: Tang, K.-W. et al . The landscape of viral expression and host gene fusion and adaptation in human cancer. Nat. Commun. 4:2513 doi: 10.1038/ncomms3513 (2013).